Sustained GSK3 activity markedly facilitates nerve regeneration Promotion of axonal growth of injured DRG neurons improves the functional recovery associated with peripheral nerve regeneration. Both isoforms of glycogen synthase kinase 3 (GSK3; α and β) are phosphorylated and inactivated via phosphatidylinositide 3-kinase (PI3K)/AKT signalling upon sciatic nerve crush (SNC). However, the role of GSK3 phosphorylation in this context is highly controversial. Here we use knock-in mice expressing GSK3 isoforms resistant to inhibitory PI3K/AKT phosphorylation, and unexpectedly find markedly accelerated axon growth of DRG neurons in culture and in vivo after SNC compared with controls. Moreover, this enhanced regeneration strikingly accelerates functional recovery after SNC. These effects are GSK3 activity dependent and associated with elevated MAP1B phosphorylation. Altogether, our data suggest that PI3K/AKT-mediated inhibitory phosphorylation of GSK3 limits the regenerative outcome after peripheral nerve injury. Therefore, suppression of this internal ‘regenerative break’ may potentially provide a new perspective for the clinical treatment of nerve injuries. In contrast to the central nervous system (CNS), injured axons in the peripheral nervous system normally regenerate and a small percentage even reconnects to their appropriate target. This successful regeneration is associated with significant, though often incomplete functional restoration [1] , [2] . Measures increasing the growth rate of regenerating axons reportedly improve the functional outcome after peripheral nerve lesion and are therefore from a clinical point of view desirable [3] . Emerging evidence points to a relevant role for glycogen synthase kinase 3 (GSK3) in peripheral nerve regeneration [4] , [5] , [6] , [7] , [8] , [9] . Both isoforms, GSK3α and GSK3β, are serine/threonine kinases sharing across species a homology of 85% (refs 7 , 10 ). They both have a high basal activity in resting cells, but are inactivated by AKT-induced phosphorylation of serine 21 (GSK3α) and serine 9 (GSK3β), respectively [4] , [11] , [12] . However, the effect attributed to GSK3 phosphorylation with regard to axon growth as well as myelin-inhibition remains controversial. Pharmacological inhibition of GSK3 reportedly improves axon regeneration in vivo by desensitizing axons towards myelin and other CNS inhibitors [5] , suggesting that GSK3β phosphorylation facilitates axon regeneration. On the other hand, other data demonstrate that GSK3 phosphorylation is involved in inhibitory processes and therefore limits the regenerative outcome [6] . Similarly, reports regarding GSK3's role in axon growth initiation are also inconsistent. Previous studies provided evidence that inactivation of GSK3 compromises axon growth [13] , [14] , [15] and that active GSK3 is favourable for axon growth during development as it phosphorylates microtubule-associated protein 1B (MAP1B), which shifts microtubules in a dynamic state that promotes axon elongation [14] , [16] . On the other hand others suggest that spatially localized inactivation of GSK3 at the distal axon is required for efficient axon elongation of DRG neurons [4] . In addition, a recent study reported that phosphatidylinositide 3-kinase (PI3K)/AKT-mediated phosphorylation of GSK3 and subsequent SMAD1 expression regulates peripheral nerve regeneration, thereby suggesting that inactivation of GSK3 by AKT is essential for switching adult DRG neurons into a regenerative state [8] . Most studies regarding the role of GSK3 in axon regeneration so far rely mainly on pharmacological manipulation of GSK3 activity. Therefore, inconsistent results may potentially be attributable to off-target effects and the use of different inhibitors. In addition, exogenous overexpression of GSK3 might induce unphysiological high levels of GSK3. To avoid these potential complications, we took advantage of GSK3α/GSK3β double knock-in mice (GSK3 S/A ) to clarify the role of GSK3 phosphorylation in peripheral nerve regeneration. In these mice, serine 21 of GSK3α and serine 9 of GSK3β are substituted by alanine, preventing GSK3 phosphorylation by AKT [17] , thereby rendering GSK3 constitutively active without changing its physiological expression level. The current study demonstrates that both GSK3 isoforms are phosphorylated PI3K/AKT pathway dependently in adult wild-type (wt) DRG neurons after axotomy. We found that global prevention of Ser21/Ser9 GSK3 phosphorylation markedly enhances axon growth of cultured DRG neurons kinase activity dependently and leads to accelerated sciatic nerve regeneration and functional recovery. Axotomy induces serine phosphorylation of GSK3α and GSK3β GSK3 is increasingly emerging as a pivotal player in peripheral nerve regeneration, but the relevance of its activity/phosphorylation with regard to axon growth induction remains highly controversial. To analyze the phosphorylation status of GSK3 in injured dorsal root ganglion (DRG) neurons, adult wild-type (wt) mice were subjected to sciatic nerve crush (SNC). As determined by immunohistochemistry, lumbar (L3, L4) DRG neurons of untreated control mice, whose axons project into the sciatic nerve [18] revealed very little phospho-S21-GSK3α (pGSK3α) and phospho-S9-GSK3β (pGSK3β) staining ( Fig. 1a ). In comparison, levels of both pGSK3α and pGSK3β were markedly increased 5 days after SNC ( Fig. 1a ). The specificity of the applied antibodies was verified by the absence of any signal in DRG from homozygous GSK3α Ser21Ala /GSK3β Ser9Ala double knock-in (GSK3 S/A ) mice, which are incapable of phosphorylating GSK3 at serines 21 and 9, respectively. This increase in pGSK3α and pGSK3β levels was confirmed by Western-blot analysis of L3/L4 DRG lysates isolated 5 days after SNC in comparison to untreated controls. Again lysates from GSK3 S/A mice were used as specificity controls and expectedly showed no signal. Elevated GSK3 phosphorylation compared with uninjured controls was not only detected in neuronal cell bodies, but also in injured sciatic nerve tissue ( Fig. 1b , Supplementary Fig. 1 ). In addition, GSK3 phosphorylation was induced in DRG neurons after dissociation-induced axotomy ( Fig. 1c ), as the numbers of pGSK3α- and pGSK3β-positive cells were significantly increased at 3 days compared with 2 h after culture preparation ( Fig. 1c , Fig. 2b ). Therefore, phosphorylation of GSK3 at serines 21 and 9, respectively, is markedly induced in adult DRG neurons upon axotomy. 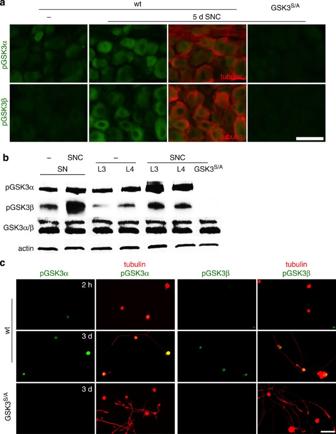Figure 1: Sciatic nerve injury induces GSK3α and GSK3β phosphorylation. (a) Immunohistochemical detection of phospho-S21-GSK3α (pGSK3α) and phospho-S9-GSK3β (pGSK3β) (green) on DRG sections from wild-type (wt) and GSK3 double knock-in mice (GSK3S/A). Animals received either no treatment (−) or a sciatic nerve crush (SNC) 5 days prior to tissue preparation. Both GSK3 isoforms were phosphorylated upon SNC in DRG neurons as detected by βIII tubulin staining (red). Scale bar, 50 μm. (b) Western-blot analysis detecting pGSK3α, pGSK3β as well as total GSK3α/β in lysates prepared from lumbar DRG (L3, L4) and sciatic nerves (SN) isolated from either untreated (−) or from animals subjected to SNC 5 days prior to tissue isolation. In contrast to total GSK3, both phosphorylated isoforms were upregulated in DRG and proximal sciatic nerve stumps upon injury. Lysates from GSK3S/Aanimals verified the specificity of the antibodies. Actin served as additional loading control. (c) Immunocytochemical staining of dissociated adult mouse DRG cultures derived from either wt or GSK3S/Atransgenic mice using antibodies against phospho-S21-GSK3α (α) or phospho-S9-GSK3β (β) (green) and βIII-tubulin (red) to detect DRG neurons. Cultures were incubated either for 2 h or 3 days as indicated. GSK3 phosphorylation was induced in dissociated adult DRG neurons. Scale bar, 50 μm. Figure 1: Sciatic nerve injury induces GSK3α and GSK3β phosphorylation. ( a ) Immunohistochemical detection of phospho-S21-GSK3α (pGSK3α) and phospho-S9-GSK3β (pGSK3β) (green) on DRG sections from wild-type (wt) and GSK3 double knock-in mice (GSK3 S/A ). Animals received either no treatment (−) or a sciatic nerve crush (SNC) 5 days prior to tissue preparation. Both GSK3 isoforms were phosphorylated upon SNC in DRG neurons as detected by βIII tubulin staining (red). Scale bar, 50 μm. ( b ) Western-blot analysis detecting pGSK3α, pGSK3β as well as total GSK3α/β in lysates prepared from lumbar DRG (L3, L4) and sciatic nerves (SN) isolated from either untreated (−) or from animals subjected to SNC 5 days prior to tissue isolation. In contrast to total GSK3, both phosphorylated isoforms were upregulated in DRG and proximal sciatic nerve stumps upon injury. Lysates from GSK3 S/A animals verified the specificity of the antibodies. Actin served as additional loading control. ( c ) Immunocytochemical staining of dissociated adult mouse DRG cultures derived from either wt or GSK3 S/A transgenic mice using antibodies against phospho-S21-GSK3α (α) or phospho-S9-GSK3β (β) (green) and βIII-tubulin (red) to detect DRG neurons. Cultures were incubated either for 2 h or 3 days as indicated. GSK3 phosphorylation was induced in dissociated adult DRG neurons. Scale bar, 50 μm. 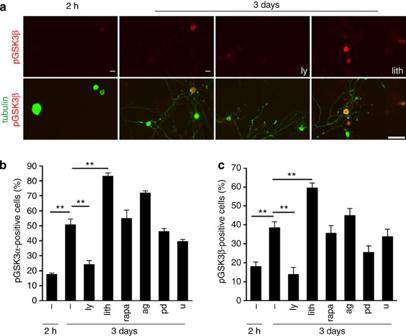Figure 2: Axotomy-induced GSK3 phosphorylation is PI3K/AKT dependent. (a) Dissociated adult DRG cultures were immunocytochemically stained for phospho-S21-GSK3β (red) and βIII-tubulin (green) after 2 h or 3 days in culture. DRG cultures had been treated with vehicle (−), PI3K inhibitor LY294002 (ly, 1 μM) or GSK3 inhibitor lithium (lith, 3 mM). Scale bar, 100 μm. (b) Quantification of pGSK3α positive DRG neurons in experimental groups as described inaand additional treatments with the mTOR inhibitor rapamycin (rapa, 10 nM), the JAK inhibitor AG490 (ag, 5 μM) and the ERK inhibitors PD98059 (pd, 5 μM) and U0126 (u, 5 μM). (c) Quantification of pGSK3β positive DRG neurons in cultures as described inb. Experiments shown ina–cwere performed three times each. The error bars represent the standard error of the mean. Statistical significance was determined with ANOVA and thepost-hocHolm Sidac test. Treatment effects: **P≤0.001. Full size image Figure 2: Axotomy-induced GSK3 phosphorylation is PI3K/AKT dependent. ( a ) Dissociated adult DRG cultures were immunocytochemically stained for phospho-S21-GSK3β (red) and βIII-tubulin (green) after 2 h or 3 days in culture. DRG cultures had been treated with vehicle (−), PI3K inhibitor LY294002 (ly, 1 μM) or GSK3 inhibitor lithium (lith, 3 mM). Scale bar, 100 μm. ( b ) Quantification of pGSK3α positive DRG neurons in experimental groups as described in a and additional treatments with the mTOR inhibitor rapamycin (rapa, 10 nM), the JAK inhibitor AG490 (ag, 5 μM) and the ERK inhibitors PD98059 (pd, 5 μM) and U0126 (u, 5 μM). ( c ) Quantification of pGSK3β positive DRG neurons in cultures as described in b . Experiments shown in a – c were performed three times each. The error bars represent the standard error of the mean. Statistical significance was determined with ANOVA and the post-hoc Holm Sidac test. Treatment effects: ** P ≤0.001. Full size image GSK3 phosphorylation depends on PI3K/AKT signalling Next we addressed the question, which signalling pathway(s) might mediate this axotomy-induced GSK3 phosphorylation. To this end, the number of pGSK3α- and pGSK3β-positive DRG neurons cultured in the presence of various signalling pathway inhibitors was determined ( Fig. 2 ). Expectedly, axotomy-induced GSK3α- and GSK3β-phosphorylation was abrogated with the PI3K/AKT inhibitor (LY294002), but not with inhibitors of mammalian Target of Rapamycin (mTOR) (rapamycin), the JAK/STAT3- (AG490) or the MAPK/ERK-signalling pathways (PD98059 and U0126) ( Fig. 2a–c ). Lithium, which induces inhibitory GSK3 phosphorylation via AKT activation and protein phosphatase-1 suppression [19] served as positive control, expectedly further increasing GSK3 phosphorylation ( Fig. 2a–c ). Prevention of GSK3 phosphorylation promotes axonal growth Previous studies suggested a requirement of GSK3 serine phosphorylation for the transformation of DRG neurons into a regenerative state [4] , [8] . We therefore compared the axon growth capacity of DRG neurons isolated from transgenic GSK3 S/A with wt mice in vitro . Surprisingly, GSK3 S/A DRG neurons showed markedly increased axonal growth in comparison to neurons from wt animals ( Fig. 3a,b ). Interestingly, growth induction was comparable for neurons from homo- and heterozygous knock-in mice. Therefore, the observed growth promotion seemed to be mediated by sustained GSK3 activity rather than the complete absence of phosphorylated GSK3. Survival of cultured DRG neurons was similar in all experimental conditions, indicating that GSK3 S/A -mediated effects were restricted to axon growth ( Supplementary Fig. 2 ). 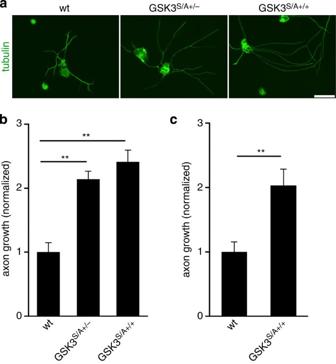Figure 3: Impediment of GSK3 phosphorylation promotes axonal growth. (a) Dissociated DRG neurons isolated from either wild-type (wt), heterozygous (GSK3S/A+/−) or homozygous (GSK3S/A+/+) GSK3αS21A/GSK3βS9Adouble knock-in mice were stained with βIII-tubulin after 2 days in culture. Scale bar, 100 μm. (b) Quantification of DRG axon growth of cultures depicted ina. Data were normalized from three independent experiments to the vehicle-treated control group with an average axon length of 193 μm per DRG neuron. Homo and heterozygous GSK3S/Aneurons show significantly increased axonal growth compared with wt controls. (c) Quantification of axon growth of adult DRG neurons from wt and double knock-in mice 20 h after replating. Data from two independent experiments were normalized to the control group with an average axon length of 21 μm per DRG neuron. The error bars inbandcrepresent the standard error of the mean. Statistical significance was determined with ANOVA and thepost-hocHolm Sidac test. Treatment effects: **P≤0.001. Figure 3: Impediment of GSK3 phosphorylation promotes axonal growth. ( a ) Dissociated DRG neurons isolated from either wild-type (wt), heterozygous (GSK3 S/A+/− ) or homozygous (GSK3 S/A+/+ ) GSK3α S21A /GSK3β S9A double knock-in mice were stained with βIII-tubulin after 2 days in culture. Scale bar, 100 μm. ( b ) Quantification of DRG axon growth of cultures depicted in a . Data were normalized from three independent experiments to the vehicle-treated control group with an average axon length of 193 μm per DRG neuron. Homo and heterozygous GSK3 S/A neurons show significantly increased axonal growth compared with wt controls. ( c ) Quantification of axon growth of adult DRG neurons from wt and double knock-in mice 20 h after replating. Data from two independent experiments were normalized to the control group with an average axon length of 21 μm per DRG neuron. The error bars in b and c represent the standard error of the mean. Statistical significance was determined with ANOVA and the post-hoc Holm Sidac test. Treatment effects: ** P ≤0.001. Full size image In addition, we tested the effect of GSK3 S/A on conditioning lesion-induced axon growth, employing a replating method described previously [8] . Therefore DRG neurons were cultured for 3 days and replated afterwards overnight ( Fig. 3c ). Similarly, axon growth from GSK3 S/A neurons was significantly stronger compared with neurons from wt animals, providing further evidence that GSK3 phosphorylation is not required for axon growth stimulation. GSK3 S/A -stimulated axon growth depends on kinase activity To test our hypothesis that GSK3 S/A -mediated axon growth promotion depends on sustained kinase activity rather than the ablation of phosphorylated GSK3, cultured DRG neurons isolated from either GSK3 S/A or wt mice were exposed to the GSK3 inhibitors lithium and SB415286 (SB), respectively ( Fig. 4 ). In contrast to lithium, SB directly blocks the substrate-binding site of GSK3 to reduce its activity instead of relying on inhibitory phosphorylation of serines 21/9 (ref. 20 ). In contrast to lithium, which did not affect the increased axon growth of GSK3 S/A DRG neurons, axon growth was significantly reduced by SB ( Fig. 4b ). These data suggest a kinase activity-dependent mechanism of GSK3 S/A for axon growth promotion. 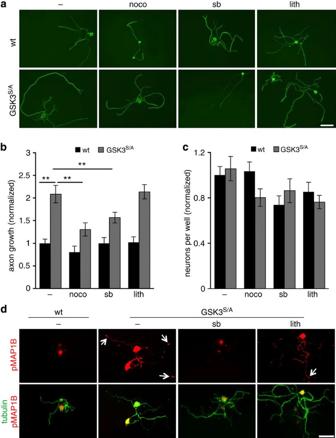Figure 4: Axon growth stimulation depends on GSK3S/Akinase activity. (a) βIII-tubulin-positive mouse DRG neurons of either wild-type (wt) or GSK3S/Amice were exposed to either vehicle (−), nocodazole (noco, 10 nM), SB415286 (sb, 5 μM) or lithium chloride (lith, 3 mM) for 2 days in culture. Scale bar, 100 μm. (b) Quantification of DRG axon growth in cultures depicted ina. Values from three independent experiments were normalized to vehicle-treated control groups with an average axon length of 143 μm per DRG neuron. Axon growth stimulation by GSK3S/Aneurons is blocked by nocodazole and SB415286, but not lithium indicating kinase activity dependence. The error bars represent the standard error of the mean. Statistical significance was determined with ANOVA and thepost-hocHolm Sidac test. Treatment effects: **P≤0.001. (c) Quantification of the number of DRG neurons for each experimental group shown ina, demonstrating similar numbers per well. Data of three independent experiments were normalized to the control group (78 DRG neurons per well). The error bars represent the standard error of the mean. (d) Dissociated adult mouse DRG cultures from either wt or GSK3S/Amice were exposed either to vehicle, lithium (lith, 3 mM) or SB415286 (sb, 5 μM) for 3 days and stained with antibodies against phospho-MAP1B (pMAP1B, red) βIII-tubulin (green). Arrows indicate axons. GSK3S/Aneurons show stronger pMAP1B staining than controls. Elevation of pMAP1B levels in GSK3S/Aneurons is blocked in the presence of SB415286, but not lithium, verifying the dependence on GSK3 activity. Scale bar, 50 μm. Figure 4: Axon growth stimulation depends on GSK3 S/A kinase activity. ( a ) βIII-tubulin-positive mouse DRG neurons of either wild-type (wt) or GSK3 S/A mice were exposed to either vehicle (−), nocodazole (noco, 10 nM), SB415286 (sb, 5 μM) or lithium chloride (lith, 3 mM) for 2 days in culture. Scale bar, 100 μm. ( b ) Quantification of DRG axon growth in cultures depicted in a . Values from three independent experiments were normalized to vehicle-treated control groups with an average axon length of 143 μm per DRG neuron. Axon growth stimulation by GSK3 S/A neurons is blocked by nocodazole and SB415286, but not lithium indicating kinase activity dependence. The error bars represent the standard error of the mean. Statistical significance was determined with ANOVA and the post-hoc Holm Sidac test. Treatment effects: ** P ≤0.001. ( c ) Quantification of the number of DRG neurons for each experimental group shown in a , demonstrating similar numbers per well. Data of three independent experiments were normalized to the control group (78 DRG neurons per well). The error bars represent the standard error of the mean. ( d ) Dissociated adult mouse DRG cultures from either wt or GSK3 S/A mice were exposed either to vehicle, lithium (lith, 3 mM) or SB415286 (sb, 5 μM) for 3 days and stained with antibodies against phospho-MAP1B (pMAP1B, red) βIII-tubulin (green). Arrows indicate axons. GSK3 S/A neurons show stronger pMAP1B staining than controls. Elevation of pMAP1B levels in GSK3 S/A neurons is blocked in the presence of SB415286, but not lithium, verifying the dependence on GSK3 activity. Scale bar, 50 μm. Full size image As GSK3 S/A might nevertheless be inactivated by an unknown mechanism, we also examined the phosphorylation levels of MAP1B, a well-known substrate of GSK3, which does not require prior priming [16] . Wt DRG cultures contained only very few neurons with pMAP1B-positive axons. In contrast, pMAP1B was detected in almost all axons of GSK3 S/A neurons, indicating robust GSK activity ( Fig. 4d ). Accordingly, MAP1B phosphorylation was blocked in the presence of the GSK3 inhibitor SB, but not lithium. GSK3 activity reportedly modulates the stability of microtubules, thereby affecting axonal growth [21] , [22] , [23] . We therefore reasoned that axonal growth of GSK3 S/A neurons might be more susceptible to microtubules-disrupting agents. To address this possibiity we exposed DRG cultures to different concentrations of nocodazole, which induces the depolymerization of microtubules. Nocodazol concentrations not affecting axonal growth of wt neurons ( Fig. 4a,b ) significantly reduced growth of GSK3 S/A neurons to comparable levels as in the wt and thereby blocking the growth-promoting GSK3 S/A effect. In conclusion, the overall beneficial effect of constitutively active GSK3 may, at least partially, be mediated by the modulation of microtubules dynamics. Effects of GSK3 phosphorylation on gene expression Transformation of injured DRG neurons into a regenerative state and associated PI3K/AKT-induced GAP43 expression has recently been reported to depend on inhibitory GSK3 serine phosphorylation [8] . We therefore investigated whether the induction of regeneration-associated-genes, such as GAP43 and SPRR1a might be affected in GSK3 S/A mice. As measured by quantitative real-time PCR, expression of both genes was strongly induced 5 days after SNC in wt as well as in GSK3 S/A mice ( Fig. 5a,b ). Consistent with our functional data, expression of GAP43 and SPRR1a was not reduced, but rather slightly elevated in GSK3 S/A compared with wt mice. Similar GAP43-protein expression of equally treated samples from GSK3 mutant and wt animals was confirmed by Western-blot analysis ( Fig. 5c ) and immunocytochemistry on cultured DRG neurons ( Fig. 5d ). 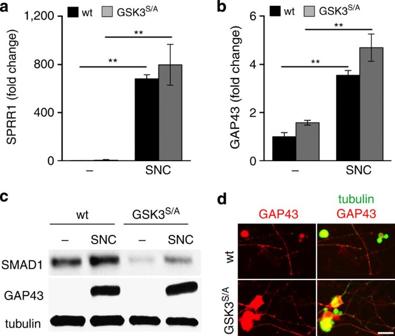Figure 5: Effect of sustained GSK3 activity on gene expression. (a,b) Quantitative real-time PCR of SPRR1a (a) and GAP43 (b) expression relative to GAPDH expression in adult DRG from either wild-type (wt) or GSK3S/Amice prior to sciatic nerve crush (—) or 5 days thereafter (SNC). Values represent means from four different animals. Error bars represent the standard error of the mean. Statistical significance was determined with ANOVA and thepost-hocHolm Sidac test. Measured treatment effects: **P≤0.001. (c) Western-blot analysis showing SMAD1 and GAP43 expression prior to SNC (−) and 5 days after SNC in wt and GSK3S/Amice. Overall expression of SMAD1 is strongly reduced in GSK3S/Amice compared with wt animals, although both genotypes show an induction of SMAD1 following SNC. GAP43-protein levels are elevated similarly after SNC in both genotypes as compared with uninjured DRG. Tubulin served as loading control. (d) Immunocytochemical staining of dissociated adult DRG neurons (detected by βIII tubulin; green) verifies similar GAP43-protein expression (red) in GSK3S/Amice compared with wt controls after 3 days in culture, scale bar, 20 μm. Figure 5: Effect of sustained GSK3 activity on gene expression. ( a , b ) Quantitative real-time PCR of SPRR1a ( a ) and GAP43 ( b ) expression relative to GAPDH expression in adult DRG from either wild-type (wt) or GSK3 S/A mice prior to sciatic nerve crush (—) or 5 days thereafter (SNC). Values represent means from four different animals. Error bars represent the standard error of the mean. Statistical significance was determined with ANOVA and the post-hoc Holm Sidac test. Measured treatment effects: ** P ≤0.001. ( c ) Western-blot analysis showing SMAD1 and GAP43 expression prior to SNC (−) and 5 days after SNC in wt and GSK3 S/A mice. Overall expression of SMAD1 is strongly reduced in GSK3 S/A mice compared with wt animals, although both genotypes show an induction of SMAD1 following SNC. GAP43-protein levels are elevated similarly after SNC in both genotypes as compared with uninjured DRG. Tubulin served as loading control. ( d ) Immunocytochemical staining of dissociated adult DRG neurons (detected by βIII tubulin; green) verifies similar GAP43-protein expression (red) in GSK3 S/A mice compared with wt controls after 3 days in culture, scale bar, 20 μm. Full size image Saijilafu et al . [8] also suggested that PI3K/AKT/GSK3 regulates axon regeneration by the induction of SMAD1 expression. We therefore analyzed the expression of this transcription factor upon SNC in GSK3 S/A animals. Consistent with Saijilafu et al . [8] , we found that the overall expression of SMAD1 was strongly reduced in GSK3 S/A mice compared with wt animals ( Fig. 5c ), verifying that the cellular presence of SMAD1 depends on GSK3 activity. However, despite the strongly reduced overall expression of SMAD1 in GSK3 S/A mice its expression was still increased by SNC, suggesting that additional mechanisms are involved in this process. Moreover, these data demonstrate that elevation of SMAD1 expression above basal levels is not essentially required for axon regeneration. Sustained GSK3 activity facilitates axonal regeneration in vivo As we observed markedly increased axonal growth of cultured GSK3 S/A DRG neurons, we next investigated the impact of GSK3 S/A on sciatic nerve regeneration in vivo . To this end, the number of SCG10-positive, regenerating axons was quantified at varying distances beyond the lesion site at 3 days after SNC. Regeneration was markedly increased particularly at longer distances in GSK3 S/A mice compared with wt controls ( Fig. 6a–d,f ). Beyond 3 mm from the lesion site, axons were only detected in GSK3 S/A , but not wt animals ( Fig. 6a–d ) indicating accelerated axonal growth. These findings were confirmed by neurofilament staining of respective sciatic nerve cross-sections at 3 mm past the crush site 3 days after injury ( Fig. 6f ). In addition, regenerating axons of GSK3 S/A mice showed a higher staining intensity for pMAP1B compared with wt animals ( Fig. 6e ), indicating an elevated GSK3 activity in regenerating axons of GSK3 S/A animals. 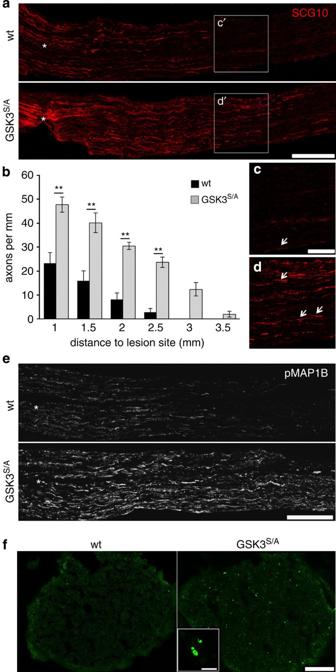Figure 6: GSK3S/Afacilitates axon regeneration in the injured sciatic nerve. (a) Longitudinal sections of sciatic nerves from wild-type (wt) and GSK3 double knock-in mice (GSK3S/A) were stained with a SCG10 antibody 3 days after injury. Scale bar, 500 μm. Asterisks indicate the crush site. (b) Quantification of SCG10 stained axons regenerating 1, 1.5, 2, 2.5, 3 and 3.5 mm beyond the lesion site 3 days after SNC. Five to eight animals were analyzed per treatment group. At least six sections per animal were analyzed. Data demonstrate significantly more regenerating axons at longer distances in the lesioned sciatic nerve of GSK3S/Acompared with wt animals. The error bars represent the standard error of the mean. Statistical significance was determined with ANOVA and thepost-hocHolm Sidac test. Treatment effects: **P≤0.001. (c,d) Higher magnification of sciatic nerve sections from wt and GSK3S/Aanimals as depicted inaapproximately 2 mm distal from the crush site. Arrows indicate single regenerating axons. Scale bar, 160 μm. (e) Longitudinal sections of sciatic nerves from wt and GSK3S/Awere stained with a phospho-MAP1B (pMAP1B) antibody 3 days after sciatic nerve crush (SNC). Levels of pMAP1B are increased in regenerating GSK3S/Aaxons. Scale bar, 500 μm. Asterisks indicate the crush site. (f) Cross-sections of sciatic nerves from wt and GSK3S/A3 mm distal to the lesion site were stained with a neurofilament antibody 3 days after sciatic nerve crush. Single axons are shown at larger magnification in the inset. Scale bar (whole nerve), 100 μm; scale bar (inset), 5 μm. Figure 6: GSK3 S/A facilitates axon regeneration in the injured sciatic nerve. ( a ) Longitudinal sections of sciatic nerves from wild-type (wt) and GSK3 double knock-in mice (GSK3 S/A ) were stained with a SCG10 antibody 3 days after injury. Scale bar, 500 μm. Asterisks indicate the crush site. ( b ) Quantification of SCG10 stained axons regenerating 1, 1.5, 2, 2.5, 3 and 3.5 mm beyond the lesion site 3 days after SNC. Five to eight animals were analyzed per treatment group. At least six sections per animal were analyzed. Data demonstrate significantly more regenerating axons at longer distances in the lesioned sciatic nerve of GSK3 S/A compared with wt animals. The error bars represent the standard error of the mean. Statistical significance was determined with ANOVA and the post-hoc Holm Sidac test. Treatment effects: ** P ≤0.001. ( c , d ) Higher magnification of sciatic nerve sections from wt and GSK3 S/A animals as depicted in a approximately 2 mm distal from the crush site. Arrows indicate single regenerating axons. Scale bar, 160 μm. ( e ) Longitudinal sections of sciatic nerves from wt and GSK3 S/A were stained with a phospho-MAP1B (pMAP1B) antibody 3 days after sciatic nerve crush (SNC). Levels of pMAP1B are increased in regenerating GSK3 S/A axons. Scale bar, 500 μm. Asterisks indicate the crush site. ( f ) Cross-sections of sciatic nerves from wt and GSK3 S/A 3 mm distal to the lesion site were stained with a neurofilament antibody 3 days after sciatic nerve crush. Single axons are shown at larger magnification in the inset. Scale bar (whole nerve), 100 μm; scale bar (inset), 5 μm. Full size image Functional recovery is accelerated in GSK3 S/A mice after SNC Motor and sensory recovery upon SNC are commonly assessed using the toe spreading and the von Frey tests, respectively [24] , [25] . Therefore, we determined the static sciatic index (SSI) in GSK3 S/A compared with wt mice [26] . No statistical differences in baseline SSI and SSI at 1 and 4 days after SNC was detected between uninjured mice ( Fig. 7a,b ). However, the SSI was significantly higher at 7–21 days after SNC in GSK3 S/A compared with wt mice, indicating improved motor function recovery ( Fig. 7a,b ). The re-establishment of neuromuscular junctions 7 days after SCN in GSK3 S/A mice was confirmed by neurofilament and α-bungarotoxin co-stainings of extensor hallucis longus (EHL) muscles. Re-established neuromuscular junctions were only found in GSK3 S/A but not in wt muscles at this time point ( Fig. 7c ). 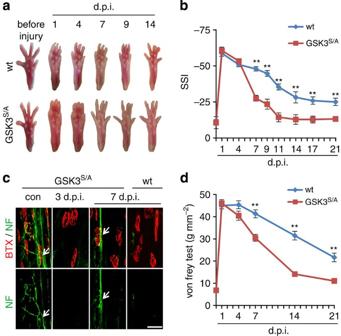Figure 7: GSK3S/Aaccelerates functional recovery upon sciatic nerve crush. (a) Representative pictures of the right hind paws of wild-type (wt) and GSK3 knock-in mice (GSK3S/A) prior to and at 1, 4, 7, 9 and 14 days post sciatic nerve crush (d.p.i.), demonstrating the improved functional recovery in GSK3S/A. (b) Quantification of functional motor recovery determined by the static sciatic index (SSI) of wt and GSK3S/Aat various days post SNC. Treatment effects: **P≤0.001. (c) α-bungarowtoxin (BTX) and neurofilament staining of extensor hallucis longus wholemounts from wt and GSK3S/Awithout injury, 3 and 7 days after SNC. White arrows indicate synapses. Re-formation of neuromuscular junctions are seen in GSK3S/Aat 7 d.p.i. (d) Sensory functional recovery determined by the von Frey test of wt and GSK3S/Aat various days after injury. Treatment effects: **P≤0.001. Figure 7: GSK3 S/A accelerates functional recovery upon sciatic nerve crush. ( a ) Representative pictures of the right hind paws of wild-type (wt) and GSK3 knock-in mice (GSK3 S/A ) prior to and at 1, 4, 7, 9 and 14 days post sciatic nerve crush (d.p.i. ), demonstrating the improved functional recovery in GSK3 S/A . ( b ) Quantification of functional motor recovery determined by the static sciatic index (SSI) of wt and GSK3 S/A at various days post SNC. Treatment effects: ** P ≤0.001. ( c ) α-bungarowtoxin (BTX) and neurofilament staining of extensor hallucis longus wholemounts from wt and GSK3 S/A without injury, 3 and 7 days after SNC. White arrows indicate synapses. Re-formation of neuromuscular junctions are seen in GSK3 S/A at 7 d.p.i. ( d ) Sensory functional recovery determined by the von Frey test of wt and GSK3 S/A at various days after injury. Treatment effects: ** P ≤0.001. Full size image Sensory recovery was measured using the von Frey test that determines the thickness of a filament required to induce a hind paw withdrawal response [25] . Uninjured wt and GSK3 S/A animals showed comparable baseline responses ( Fig. 7d ). The required force markedly increased to a similar extent in both groups at 1 day after SNC, indicating a dramatic loss of touch sensation after SNC. Animals started to recover touch sensation 7 days after injury and continued over a time period of 21 days with GSK3 S/A animals improving significantly faster than wt animals at all time points analyzed ( Fig. 7d ). In summary, these data demonstrate that increased axon growth was associated with accelerated functional recovery upon injury. The current study investigated the role of AKT-mediated inhibitory GSK3 phosphorylation in adult peripheral nerve regeneration. Surprisingly, maintained GSK3 activity in GSK3 S/A neurons markedly promoted axon regeneration and accelerated functional recovery after peripheral nerve injury in adult mice. These findings reveal an unexpected and new role of GSK3 in this context and are potentially meaningful for the development of novel therapies for peripheral nerve injury. The essential role of the PI3K/AKT signalling pathway in stimulating axon regenerative processes in the adult central and peripheral nervous systems is well documented [8] , [27] , [28] , [29] , [30] . Activated AKT phosphorylates GSK3α at serine 21 (pGSK3α) and GSK3β at serine 9 (pGSK3β) and thereby inhibits their respective kinase activity [7] , [31] , [32] . Consistent with elevated PI3/AKT activity in DRG neurons upon peripheral nerve injury [8] , the current study found a robust increase of pGSK3α and pGSK3β levels in DRG neurons and the proximal sciatic nerve upon SNC. In addition, DRG neurons also increased pGSK3 levels after a few hours in culture, most likely due to the axotomy associated with tissue dissociation. Inhibition of GSK3 phosphorylation in the presence of a PI3K inhibitor confirmed the dependence of this process on the PI3K/AKT signalling pathway. A previous report suggested that inhibitory phosphorylation of GSK3s is essentially required for transforming DRG neurons into a regenerative state and therefore for axon regeneration upon injury in general [8] . This notion is mainly based on observations that the inhibitory effect of a PI3K inhibitor on axon growth of cultured DRG neurons was rescued in the presence of pharmacological GSK3 inhibitors [8] . However, some of these inhibitors show low selectivity and high IC 50 values potentially affecting other structurally similar kinases [33] , [34] . Complementary supportive experiments testing whether genetically modified GSK3 without the inhibitory GSK3-phosphorylation site would compromise axon growth were not performed. To address this point in our study, we used well-established GSK3 double knock-in mice, which are globally resistant to AKT-mediated GSK3 phosphorylation at serine 21/9 (refs 17 , 35 ). Instead of the expected decrease, axon regeneration in cell culture and in vivo was markedly improved in GSK3 S/A neurons compared with controls even when the neurons were primed after replating. Moreover, induction of the regeneration-associated genes GAP43 and SPRR1A upon SNC was not compromised in GSK3 S/A animals, but rather slightly increased. Therefore, our data suggest that (1) GSK3 phosphorylation is not essentially required for the induction of GAP43 expression or the transformation of adult DRG neurons into a regenerative state and (2) PI3K/AKT-mediated GSK3 phosphorylation partially limits peripheral nerve regeneration. In addition, our data indicate that the observed axon growth-promoting effect depends on an overall higher kinase activity in non-phosphorylatable GSK3 S/A neurons. The presence of SB415286, a competitive inhibitor directly blocking the substrate-binding site of GSK3 (ref. 20 ), specifically abrogated increased axonal growth, while lithium, a non-competitive inhibitor impeding GSK3 activity via S21/9 phosphorylation, showed no effect on GSK3 S/A neurons. Together with the observation that direct phosphorylation of MAP1B at Th1265 by GSK3, which does not require prior priming by other kinases [16] , [22] , [36] , was significantly elevated in neurons of double knock-in mice, these data reflect an overall higher kinase activity of GSK3 S/A compared with controls. Moreover, these data exclude the inhibition of the GSK3 kinase activity by another, unknown compensatory mechanism in GSK3 S/A mice. This idea is also supported by the strong reduction of SMAD1 expression in GSK3 S/A compared with wt DRG, as neuronal SMAD1 expression levels are regulated by GSK3 activity [8] . However, as axon regeneration was promoted in GSK3 S/A mice, these data demonstrate that elevation of SMAD1 expression above basal levels in wt animals is not required for the transformation of DRG neurons into a regenerative state, without excluding the possibility that basal SMAD1 levels are essential for axon growth [37] . Interestingly, despite the overall strong reduction of SMAD1 expression in GSK3 S/A mice, expression of this transcription factor was still increased after SNC in these animals, demonstrating GSK3 phosphorylation-independent upregulation. Altogether these data do not support the concept that PI3K-GSK3 signalling mainly regulates axon regeneration by inducing the expression of Smad1 as recently stated by others [8] . To our knowledge this is the first report showing that maintenance of GSK3 activity facilitates axon regeneration in the adult nervous system. In the developing nervous system, GSK3 regulates the activity of several microtubule associated proteins (MAPs) [4] , [13] , [21] , [22] , [23] , [38] , [39] and thereby controls directed growth cone advancement and guidance. One of these proteins is MAP1B, which is required for axon growth [40] . MAP1B exists in at least two different modes of phosphorylation [41] , with mode II phosphorylation being mediated mainly by casein kinase II (refs 41 , 42 ) and occurring throughout the whole neuron. In contrast, mode I phosphorylation of MAP1B is concentrated in the distal part of the axon [43] and switches microtubules into a dynamic state by promoting tyrosination of α-tubulin [40] , [44] . Active GSK3 has been described to mediate this mode I phosphorylation at the two non-primed sites Serine 1,260 and Threonine 1,265 (refs 14 , 22 , 36 ). Decreased MAP1B mode I phosphorylation evoked by the application of GSK3 inhibitors reportedly reduces axon growth of embryonic chick DRG explants [13] and dissociated cultures [6] , [39] . Moreover, GSK3-mediated phosphorylation of MAP1B compromises the detyrosination of microtubules, thereby keeping microtubules in a dynamically unstable state. This renders them more sensitive to nocodazole depolymerization, but also facilitates axon growth in embryonic tissue [13] , [16] . As demonstrated by the current study, non-primed MAP1B phosphorylation by GSK3 is increased in adult neurons of GSK3 S/A mice, and low concentrations of nocodazole specifically abolish the axon growth-promoting effect in GSK3 S/A , while wt neurons were not affected ( Fig. 4b ). Therefore, these data support the notion that GSK3 S/A promotes axon growth, at least partially, via pMAP1B-dependent modulation of microtubules dynamics. Further investigations are required to address this possibility directly. Beside the modulation of growth cone dynamics, constitutive GSK3 activity could affect the expression of regeneration-associated genes, thereby elevating the intrinsic growth state of the DRG neurons. GSK3 is known to interact with several transcription factors involved in axon growth [45] , [46] , [47] . Albeit the underlying mechanism, maintaining GSK3 activity in GSK3 S/A mice significantly accelerated axon regeneration in the injured sciatic nerve in vivo compared with wt mice. In GSK3 S/A mice the number of axons at 3 mm beyond the lesion site was comparable to the number found at 1.5 mm in wt animals 3 days after injury, and re-established neuromuscular junctions in the EHL were only detected in GSK3 S/A mice after 7 days. Consistent with the increased axonal growth observed in cell culture these data demonstrate that GSK3 S/A markedly promotes axonal regeneration in vivo and accelerates functional recovery, as indicated by sensory and motor behavioural tests of GSK3 S/A mice, compared with wt animals. Therefore, therapies specifically preventing GSK3 phosphorylation without affecting PI3K activity, for instance by drugs or gene therapy, may constitute useful treatments to improve peripheral nerve regeneration. Future experiments will reveal whether the beneficial effects of constitutively active GSK3 seen in the current study are also applicable to CNS regeneration. Surgical procedures All animal protocols were approved by the local authorities and adhered to the respective animal care guidelines (Regierungspräsidium Recklinghausen). SNC was performed as described previously [48] . In brief, male and female adult (8–12 weeks) wt, homo and heterozygous GSK3α S21A /GSK3β S9A mice were maintained on a 12-h light/dark cycle with ad libitum access to food and water. Animals were housed under the same conditions for at least 10 days prior to use in experiments. Animals were anesthetized by intraperitoneal injections of ketamine (60–80 mg kg −1 , Pfizer, New York, NY, USA) and xylazine (10–15 mg kg −1 , Bayer, Leverkusen, Germany). A skin incision of about 10 mm was made over the gluteal region exposing the right sciatic nerve from the sciatic notch to the point of trifurcation. The ischiocrural musculature was carefully spread minimizing tissue damage. The crush injury was performed proximal to the tibial and peroneal divisions for 30 s using a Dumont #5 forceps (Hermle, Tuttlingen, Germany) and marked with carbon (Sigma). The skin was sutured afterwards. The left sciatic nerve was left intact and served as untreated control, as indicated. DRG neuron cultures and immunocytochemical staining procedure DRG neurons were isolated from wt and homo and heterozygous GSK3α S21A /GSK3β S9A as described previously [49] . DRG (T8-L6) were harvested, incubated in 0.25% trypsin/EDTA (GE Healthcare, Chalfont St Giles, UK) and 0.3% collagenase type IA (Sigma, St Louis, MO, USA) in DMEM (Life Technologies, Carlsbad, CA, USA) at 37 °C and 5% CO 2 for 45 min and mechanically dissociated. Cells were resuspended in DMEM containing 10% foetal bovine serum (GE Healthcare) penicillin/streptomycin (500 U ml −1 ; Merck Millipore, Billerica, MA, USA) and 5-fluoro-2′-desoxyuridine (100 nM; Sigma). Cells were cultured on poly-D-lysine (0.1 mg ml −1 , molecular weight <300,000 kDa; Sigma) and laminin (20 μg ml −1 ; Sigma) coated 96 well plates (Nunc, Germany) at 37 °C and 5% CO 2 . To test the effect of sustained GSK3 activity on axonal growth, dissociated DRG neurons from wt and GSK3 S/A mice were cultured for 48 h. Cells were then fixed with 4% paraformaldehyde (PFA; Sigma) and immunocytochemically stained with antibodies against 200 kDa neurofilament heavy chain (1:2,000; ab8135, Abcam, Cambridge, UK) and βIII-tubulin (1:2,000; Covance, Princeton, NJ, USA). Imaging and quantification of total axon length and neuron numbers per well were automatically performed with the Pathway 855 microscope system (BD, Franklin Lakes, NJ, USA) and Attovision software, avoiding bias of quantification. Average axon length per neuron and neuron counts per group were normalized to control groups as indicated. Data are presented as the mean±s.e.m. of six replicate wells from three separate experiments. Significances of intergroup differences were evaluated using either one- or two-way analysis of variance (ANOVA) followed by Holm-Sidak post-hoc test. To assess the effect of GSK3 S/A on transcription-dependent axon growth as shown by Saijilafu et al . [8] , a replating method was employed as previously described. To this end DRG neurons were cultured for 3 days and then resuspended and replated on poly-D-lysine and laminin-coated culture dishes. After 20 h cells were fixed and immunohistochemically stained. Axonal growth was evaluated as described above. To characterize the effect of various signalling pathways upon GSK3 phosphorylation in vitro , the following signalling pathway inhibitors were added to dissociated DRG cultures: Janus kinase 2 inhibitor AG490 (5 μM, Merck Millipore), PI3k inhibitor LY294002 (1 μM, Sigma), mTOR inhibitor rapamycin (10 nM, LC-Laboratories, Woburn, MA, USA), mitogen-activated protein kinase inhibitors PD98059 and U0126 (both 5 μM, Merck Millipore) and GSK3 inhibitors Lithium (3 mM, Sigma) as well as SB415286 (5 μM, Sigma). Cells were cultured for either 2 h or 3 days prior to fixation with 4% PFA and immunocytochemically stained with antibodies against phospho-S9-GSK3β (1:500; Cell Signaling, Danvers, MA, USA), phospho-S21-GSK3α (1:500, Tebu-bio, Le-Perray-en-Yvelines, France), βIII-tubulin (1:2,000; Covance), GAP43 (1:500, Invitrogen, Carlsbad, CA, USA) and pMAP1B (1:500; Thr1265; Thermo Scientific, Waltham, MA, USA). Secondary antibodies were anti-mouse immunoglobulin G (IgG) and anti-rabbit IgG antibodies conjugated to either Alexa Fluor 488 or Alexa Fluor 594 (all 1:1,000; Molecular Probes, Eugene, OR, USA). Stained DRG neurons were analyzed via fluorescence microscopy (Zeiss STX). Data are represented as normalized means ±s.e.m. from three separate experiments. Western-blot assays DRG (L3, L4) from four mice per experimental group were dissected and combined in 100 μl lysis buffer (20 mM Tris HCl pH 7.5, 10 mM KCl, 250 mM sucrose, 10 mM NaF, 1 mM DTT, 0.1 mM Na 3 VO 4 , 1% TritonX-100, 0.1% SDS and protease inhibitors; Merck Millipore). DRG were homogenized by sonification and centrifuged at 8,000 g for 10 min at 4 °C. Proteins in DRG lysates were separated by 10% SDS-polyacrylamide gel electrophoresis according to standard protocols. Proteins were then transferred to nitrocellulose membranes (Bio-Rad, Hercules, CA, USA). Blots were blocked either in 5% dried milk or 5% bovine serum albumin (Sigma) and incubated with either a monoclonal antibody against β-actin (1:7,500; Sigma), βIII-tubulin (1:2,000; Covance), SMAD1 (1:1,000; Cell Signaling), phospho-S21-GSK3α (1:2,000; Cell Signaling), phospho-S9-GSK3β (1:2,000; Cell Signaling), total GSK3α/GSK3β (1:500, Cell Signaling) or polyclonal antibodies against GAP43 (1:1,000; Invitrogen) at 4 °C overnight. All antibodies except phospho-S21-GSK3α were visualized with anti-rabbit or anti-mouse immunoglobulin G (IgG) secondary antibodies conjugated to horseradish peroxidase (1:80,000; Sigma). Phospho-S21-GSK3α antibody was recognized with a horseradish peroxidase-conjugated anti-rabbit antibody (1:4.000; Cell Signaling). Antigen–antibody complexes were visualized using enhanced chemiluminescence substrate (Bio-Rad, Hercules, CA, USA). Western-blots were repeated at least twice to verify results. Immunohistochemistry Animals were killed by cervical dislocation either immediately, or 3 or 5 days after SNC. L3 and L4 DRG and sciatic nerves were isolated, post fixed for 6 h, transferred to 30% sucrose overnight (4 °C) and embedded in Tissue-Tek (Sakura, Netherlands, Leiden). Longitudinal and cross-sections of sciatic nerves and DRG were cut on a cryostat (Leica, Wetzlar, Germany), thaw-mounted onto coated glass slides (Superfrost plus, Fisher, Pittsburgh, PA, USA) and stored at −20 °C until further use. Monoclonal antibodies against βIII-tubulin (1:2,000; Convance), phospho-S21-GSK3α (1:500; Tebu-bio, Offenbach, Germany) and phospho-S9-GSK3β (1:1,000; Cell Signaling) were used. Secondary antibodies included anti-mouse IgG and anti-rabbit IgG antibodies conjugated to either Alexa Fluor 488 or Alexa Fluor 594 (all 1:1,000; Invitrogen). Sections were embedded in Mowiol and analyzed using fluorescent microscopy. At least four animals per group were evaluated. To analyze re-establishment of neuromuscular junctions, mice were killed at 3 and 7 days after SNC. The EHL muscle was dissected and post fixed in PFA for 1 h. Afterwards muscles were permeabilized in 2% TritonX in PBS overnight. Axons where labelled with an antibody against neurofilament (1:2,000; Abcam). Synapses were visualized by incubation with α-bungarotoxin conjugated to Alexa594 (1:1,000; Invitrogen) in PBS-Tween 20 for 1 h. RNA isolation and quantitative real-time PCR For quantitative real-time PCR, DRG (L3, L4) from four mice per group were dissected and combined. Total RNA was isolated using the RNeasy mini kit (Qiagen, Hilden, Germany) according to the manufacturer’s protocol. Total RNA (40 ng) was reverse transcribed using the Superscript II reverse transcriptase kit (Invitrogen). GAP43, SPRR1a and GAPDH expression was quantified using SYBR Green PCR Master Mix (Applied Biosystems, Foster City, CA, USA) and QuantiTect primers (MmGAP43_1_SG, Mm_Gapdh_3_SG, Mm_Sprr1a_2_SG; QuantiTect Primer Assay, Qiagen) on an Applied Biosystems 7,500 real-time PCR system (Life Technologies) using 50 amplification cycles according to the manufacturer’s protocol. All reactions were performed in duplicate, and four independent samples from different mice were analyzed per experimental group. The specificity of the PCR product was verified with the dissociation curve analysis feature. Quantification of regenerating axons in the sciatic nerve Longitudinal cryosections (14 μm) of sciatic nerves were immunohistochemically stained with an antibody against the regeneration-associated protein SCG10 (Novus Biologicals, Cambridge, UK) [50] or against pMAP1B (Thermo Scientific). SCG10-positive axons were quantified at 1, 1.5, 2, 2.5, 3, 3.5 mm beyond the carbon-labelled injury site, as described previously [3] . Statistical significances of intergroup differences were evaluated using a one-way ANOVA followed by the Holm-Sidak post-hoc test. Each experimental group included at least six sections from five different mice. Static sciatic index Functional motor recovery of 15 GSK3 S/A and 13 wt mice after SNC was determined by calculating the SSI as described previously [24] , [51] . Mice were lifted from the ground to photograph the left and right hind paws, respectively. Toe spreading on the contra- (C, left) and ipsilateral (I, right) sides of the SNC was assessed in wt and transgenic GSK3 knock-in mice at 0, 1, 4, 7, 9, 11, 14, 17 and 21 days after SNC, by measuring the paw length (PL) and the distance between the first and the fifth toe (FF). The SSI was calculated based on the previously described formula [24] : SSI=101.3 ((IFF-CFF)/CFF)−54.03((IPL-CPL)/CPL)−9.5. Data are represented as mean±s.e.m. from 13–15 animals per experimental group. Statistical significances of intergroup differences were evaluated using a two-way ANOVA followed by the Holm-Sidak post-hoc test. Von frey test Functional sensory recovery after SNC was determined with the von Frey filament test as described previously [25] at 0, 1, 4, 7, 14 and 21 days after SNC in 15 GSK3 S/A and 13 wt mice. The test was performed at the same time of the day and by the same experimenter. To this end, mice were placed on an elevated metal grid (grid size: 2 mm) and allowed to acclimate for 15 min before testing. Then, responses of the ipsilateral hind paw to a range of innocuous von Frey filaments (Muromachi Kikai Co., LTD, Tokyo, Japan) were considered, starting with the smallest filament and increasing filament size until a positive response was initiated, which is indicated by a sharp withdrawal of the paw. Statistical significances of intergroup differences were evaluated using a two-way ANOVA followed by the Holm-Sidak post-hoc test. How to cite this article: Gobrecht, P. et al . Sustained GSK3 activity markedly facilitates nerve regeneration. Nat. Commun. 5:4561 doi: 10.1038/ncomms5561 (2014).